The simple fly larval visual system can process complex images Animals that have simple eyes are thought to only detect crude visual detail such as light level. However, predatory insect larvae using a small number of visual inputs seem to distinguish complex image targets. Here we show that Drosophila melanogaster larvae, which have 12 photoreceptor cells per hemisphere, are attracted to distinct motions of other, tethered larvae and that this recognition requires the visual system but not the olfactory system. In addition, attraction to tethered larvae still occurs across a clear plastic barrier, does not occur significantly in the dark and attraction occurs to a computer screen movie of larval motion. By altering the artificial attractant movie, we conclude that visual recognition involves both spatial and temporal components. Our results demonstrate that a simple but experimentally tractable visual system can distinguish complex images and that processing in the relatively large central brain may compensate for the simple input. The visual system represents a substantial source of sensory input, but in order to provide adequately processed spatial information, a two-dimensional pixel array has to be analysed. Obtaining a full image is generally achieved by using a retina with a complete two-dimensional photoreceptor set or by scanning a retinal strip across the field of view. The latter approach, used by the mantis shrimp, jumping spiders and certain molluscs [1] , requires an unusual amount of processing in order to integrate visual input with changing retinal position. Certain insect larvae, such as diving beetle larvae, also have a small number of photoreceptors and are thought to use head sweeps to scan the visual field [2] . A third potential scanning approach might hypothetically use a single or small number of visual units that would have to scan in multiple directions in order to generate an image. Such an approach would also require significant processing in order to integrate an image with photoreceptor position. Here, we demonstrate that Drosophila larvae employ a small number of visual units to discriminate complex images by employing integrated complex head sweeps or some other novel form of visual processing. Attraction can be measured in larvae using a simple assay In developing a simple locomotor plasticity assay, we found that small pieces of plastic superglued to one side of a Drosophila third instar foraging larva caused not only a temporary imbalance in locomotion but also a short-lived, writhing-like motion ( Supplementary Movie 1 ). Animals with attached plastic feed normally and shed the plastic upon the end of pupation. It was also observed that writhing larvae tend to attract neighbouring larvae that often engage in cowrithing ( Supplementary Movie 2 ). We sought to identify the nature of the attracting signal and so developed a simple assay in which three Canton S larvae (the targets) were glued to a single point on the lid of a plastic 100-mm Petri dish and the behaviour of a single, mobile larva (test larva) located on a moist surface on the floor of the dish was monitored. An attractant score was developed by examining where the test larva moved in the presence of either live or freeze-killed target larvae tethered above ( Fig. 1 ; Supplementary Fig. S1 ). The positions of the mobile larvae were determined every 30 s during a 30-min test period. Cumulative statistics from 20 individual experiments were plotted as either number of entries into ‘crossovers’ ( Fig. 1b ) or time spent in each 1/2 cm 2 of a grid overlaid on the testing chamber ( Supplementary Fig. S1a ). When compared with the average for all 1/2 cm 2 , larvae are attracted to the square under the live tethered target, but not the dead equivalent. Larvae were also ‘attracted’ to the central drop-off point, potentially owing to the deposition of trace amounts of yeast from the cuticle when the test larva was introduced into the chamber. These results cannot be explained by differences in individual locomotion as test larvae in both scenarios (with live and dead targets) travel about the same distance over the 30-min test period ( Supplementary Fig. S1c ). 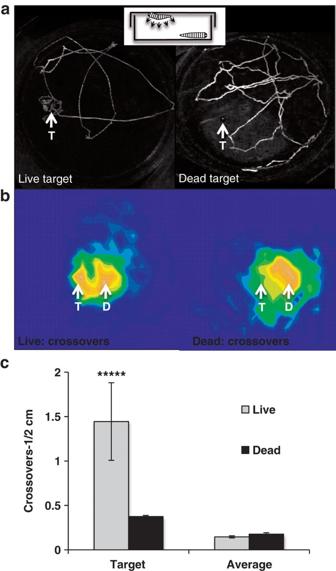Figure 1: An attraction assay forDrosophilalarvae. (a) Representative tracks ofD. melanogasterCanton S larvae in a 100 mm Petri dish after a 30-min span with either live or dead larval targets attached to the lid. ‘T’ represents the point where the target larvae are attached. (b) Cumulative plots of 20 tracks each measured as crossovers per 1/2 cm2. ‘D’ represents the drop-off point of the larvae and ‘T’ represents the tethered target larvae. (c) Counts of crossovers either averaged for just under the target or all 1/2 cm2in the 100 mm Petri dish field. Columns represent average and s.e., and significance (*****P<0.0001) represents a comparison between values under the target with the general average for that experiment using Tukey’s analysis of variance method. Figure 1: An attraction assay for Drosophila larvae. ( a ) Representative tracks of D. melanogaster Canton S larvae in a 100 mm Petri dish after a 30-min span with either live or dead larval targets attached to the lid. ‘T’ represents the point where the target larvae are attached. ( b ) Cumulative plots of 20 tracks each measured as crossovers per 1/2 cm 2 . ‘D’ represents the drop-off point of the larvae and ‘T’ represents the tethered target larvae. ( c ) Counts of crossovers either averaged for just under the target or all 1/2 cm 2 in the 100 mm Petri dish field. Columns represent average and s.e., and significance (***** P <0.0001) represents a comparison between values under the target with the general average for that experiment using Tukey’s analysis of variance method. Full size image We chose to simplify the attraction assay to measure the number of crossovers into a 1 cm square at the target so as to be able to examine a larger number of variables ( Fig. 2 ). As negative and positive controls, a glued piece of plastic (blank) and plastic with yeast paste (yeast) were used, respectively. Test larvae crossed beneath the yeast significantly more times than the blank ( Fig. 2 ; Supplementary Movies 3, 4 ). Test larvae also crossed under live tethered larvae as often as they crossed under the yeast-positive control and significantly more than the blank control ( Fig. 2 ; Supplementary Movie 5 ). Dead tethered larvae did not attract test larvae ( Fig. 2 ; Supplementary Movie 6 ). In these experiments, the attraction assay with live larvae was first conducted followed by freeze killing the attracting larvae and repeating the assay with this dead control. Dead larvae were removed from the lid after the assay, the lid was washed and a 1 × 1 mm 2 piece of white plastic was glued down to the previous glue spot as a further negative control. Finally, yeast was placed on the plastic and retested as a positive control. Thus, the position of the attractants on the lid and the matched controls was preserved. We conclude from this experiment that live tethered larvae emit an attractant signal that can be behaviourally quantified. 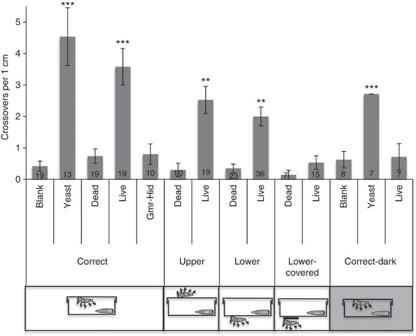Figure 2: Larvae are visually attracted to the target. Response of larvae to other tethered larvae, alive or dead, that are placed in various adjoining chambers. The first set (correct) is the same experiment as described inFig. 1. Tethered larvae are on the lid of the Petri dish in the same chamber as the test larva. In the second set, upper, the tethered larvae are on the upper lid but inverted with respect to the test larva. In the ‘lower’ set, the target larvae are tethered under the Petri dish and ‘lower-covered’ have a square of foil placed between the animals and the plastic. The last set, correct-dark, are configured the same as the ‘correct’ group except that experiments were conducted in complete darkness with an infrared camera and light recording activity. All larvae are Canton S except for ‘GMR-Hid,’ where the test larvae have Bolwig’s visual organ removed using directed expression of the Hid protein. ‘Blank’ is a piece of plastic or putty about the size of a larva and ‘yeast’ is a pellet of food yeast. Columns represent average and s.e. Numbers in the bars represent the number of independent experiments. Significance (**P<0.01; ***P<0.001) represents a comparison with ‘blank’ using Tukey’s analysis of variance method. Figure 2: Larvae are visually attracted to the target. Response of larvae to other tethered larvae, alive or dead, that are placed in various adjoining chambers. The first set (correct) is the same experiment as described in Fig. 1 . Tethered larvae are on the lid of the Petri dish in the same chamber as the test larva. In the second set, upper, the tethered larvae are on the upper lid but inverted with respect to the test larva. In the ‘lower’ set, the target larvae are tethered under the Petri dish and ‘lower-covered’ have a square of foil placed between the animals and the plastic. The last set, correct-dark, are configured the same as the ‘correct’ group except that experiments were conducted in complete darkness with an infrared camera and light recording activity. All larvae are Canton S except for ‘GMR-Hid,’ where the test larvae have Bolwig’s visual organ removed using directed expression of the Hid protein. ‘Blank’ is a piece of plastic or putty about the size of a larva and ‘yeast’ is a pellet of food yeast. Columns represent average and s.e. Numbers in the bars represent the number of independent experiments. Significance (** P <0.01; *** P <0.001) represents a comparison with ‘blank’ using Tukey’s analysis of variance method. Full size image Visual attraction in larvae requires Bolwig’s organ Chemoattractive cues likely drive larval aggregation during cooperative burrowing [3] . Therefore, we tested the ability of olfactory mutant ( or83b 1 ) [4] larvae to respond to live targets. or83b 1 larvae are not attracted to yeast (0.1±0.1, n =10). Surprisingly, or83b 1 larvae were still attracted to live tethered larvae (2.3±0.6, n =11, P <0.001), so we also tested eyeless 2 ( ey 2 ) larvae [5] and larvae rendered blind by genetic ablation of photoreceptors ( GMR-Hid ) [6] . Blind test larvae were not attracted to the live target ( Fig. 2 , data for ey 2 0.7±0.2 n =15). However, body-wall-based light sensing neurons are not required, as larvae in which these cells are ablated using Gr28b-GAL4- driven Hid are still attracted (1.9±0.3 n =18, P <0.01) [6] . This indicates that the attraction is based on visual cues obtained by photoreceptors of the larval eye, or Bolwig’s organ. To further investigate the modality responsible for attraction, we altered the placement of the target larvae as either inverted on the lid, upper, or under a propped-up dish, lower. The rationale was that while an odour attractant may still be able to enter into the Petri dish from larvae tethered outside the test chamber, it should lose positional information. As visual recognition should still occur through the plastic, this potential was blocked by placing foil between the ‘lower’ tethered larvae and the plastic chamber. With the exception of the foil-overlaid targets, all demonstrated attraction to the live target ( Fig. 2 and Supplementary Movie 7 ). Dead target controls were used for each of these three scenarios and none attracted the test larvae. To test this further, assays were also conducted in the dark using the original configuration (as shown in Fig. 1 ). We found no significant difference between the live and blank groups, while yeast still attracts in the dark ( Fig. 2 ; Supplementary Movies 8, 9, 10 ). Taken together, these experiments indicate that the attraction of individual, mobile larvae to tethered, writhing larvae is mediated through vision. Image recognition in larvae requires spatial and temporal cues If Drosophila larvae can visually recognize each other, we reasoned that video playback of a tethered larva should act as an attractant ( Supplementary Movie 11 ), providing a platform to dissect the essential components of the visual cues. We used the same arrangement as shown in Fig. 2 (lower), except an LCD screen replaced the live larvae. Using the same analysis as that described for Fig. 1 , we used three types of movie targets: a direct playback of previously recorded live tethered larvae (30 Hz), a substantially slowed playback (0.1 Hz) and a playback where resolution was decreased until target larvae only appeared as a white square of the same average luminescence as the other test movies (white square movie). Crossovers and time spent were assembled for each 1/2 cm 2 in 20 individual experiments per playback type. Only the movie playing at life-like speed (30 Hz) showed attraction measured either as time spent or crossovers ( Fig. 3 ; Supplementary Movies 12, 13 ). As in the live tethered experiments, attraction to the drop-off zone can be seen in the cumulative tracks ( Fig. 1b ; Supplementary Fig. S1a , Fig. 3 ). Again, average total distance travelled was the same for all three cases (30 Hz 60±4 mm, 0.1 Hz 49±4 mm, white square 52±6 mm). The ability of a video playback to attract individual mobile larvae provides further evidence that attraction in this assay relies on visual input. 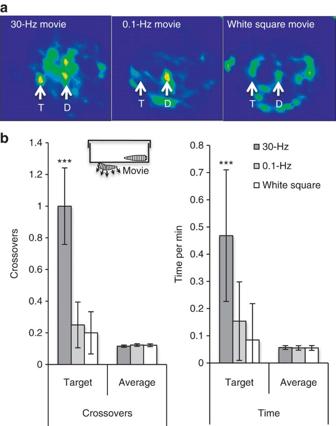Figure 3: Larvae are attracted to a movie target. (a) Cumulative tracks of 20 Canton S larvae each, crawling in a Petri dish placed over an LCD screen playing a QuickTime movie of three writhing tethered larvae. The movie was recorded at 30 Hz and replayed at true speed, 30 Hz, or 300 times more slowly, 0.1 Hz. The 1/2 cm2around the target larvae in the movie was binned such that it appears as a square with the same average lumination as the original movie but no detail, white square movie. ‘T’ is where the target movie is playing under the Petri dish, and ‘D’ is the drop-off point for the test larva. (b) Plots showing average and s.e.m. showing either crossover events or time spent per 1/2 cm2. Shown is either the crossovers or time spent in the target square, target, or averaged for all squares, average. Columns represent average and s.e. Significance (***P<0.001) represents a comparison with averaged values using Tukey’s analysis of variance method. Figure 3: Larvae are attracted to a movie target. ( a ) Cumulative tracks of 20 Canton S larvae each, crawling in a Petri dish placed over an LCD screen playing a QuickTime movie of three writhing tethered larvae. The movie was recorded at 30 Hz and replayed at true speed, 30 Hz, or 300 times more slowly, 0.1 Hz. The 1/2 cm 2 around the target larvae in the movie was binned such that it appears as a square with the same average lumination as the original movie but no detail, white square movie. ‘T’ is where the target movie is playing under the Petri dish, and ‘D’ is the drop-off point for the test larva. ( b ) Plots showing average and s.e.m. showing either crossover events or time spent per 1/2 cm 2 . Shown is either the crossovers or time spent in the target square, target, or averaged for all squares, average. Columns represent average and s.e. Significance (*** P <0.001) represents a comparison with averaged values using Tukey’s analysis of variance method. Full size image Assuming that attraction to the video target employs the same features as attraction to a live target, we sought to determine whether spatial and/or temporal cues are necessary. To test temporal features, the movie was replayed at various speeds, from 1/300 × (same as 0.1 Hz in Fig. 3 ) to 2 × , twice the normal speed ( Fig. 4 , ‘Movie speed’). This yielded a tuning curve centred on the life-like playback rate, indicating that larval processing uses temporal features of the visual stimulus. We further tested temporal resolution ( Fig. 4 , ‘temporal resolution’) by removing successive frames and playing the movie more slowly. For the 1/5 × reduction, four of every five successive frames were deleted and the subsequent movie was played at 1/5 the normal speed. This results in a movie with the normal resolution and normal movements, but abrupt changes between frames. 1/5 × and 1/50 × reduced movies failed to attract test larvae. To test spatial resolution, the movie was binned over a range from the 8-bit original (‘1 × ’ in ‘Movie speed’ group) to 40 × 40 (same as the ‘white square movie’ in Fig. 3 ). Average binning was used so that the average luminescence was the same for each square, as was movement, but edges and shapes become blurred. While 2 × 2 binning showed some attraction, further loss in spatial resolution removed the cue. Therefore, spatial cues of the visual image are also necessary. Finally, we examined whether reversing the movie (reverse), a blank screen (black), and playing frames in random order (random) solicited any attraction. Only movies played in reverse showed attraction, indicating that whatever the spatial and temporal cues, they are symmetrical in time. 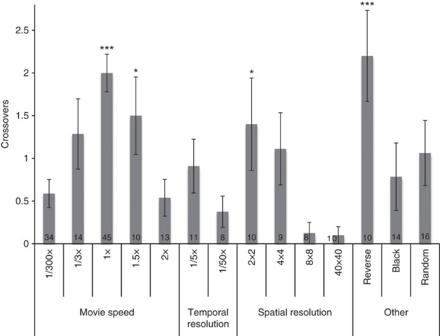Figure 4: Larvae are visually attracted via temporal and spatial cues. Averaged crossover values of Canton S larvae crawling in a Petri dish placed over an iPad 1 playing a QuickTime movie under variable conditions. Altered movie speed, Movie speed, is from 2 × (movie recorded at 30 Hz and replayed at 60 Hz) to 1/300 × , or replayed at 0.1 Hz. The test movie was average binned, spatial resolution, down to 40 × 40, which is the same as the ‘white square movie’ inFig. 3. Frames were removed, temporal resolution, either every four out of five frames, 1/5 × , or every 49 out of 50, 1/50 × , and the movie was then slowed appropriately to match the live speed. In ‘other’, the movie was either played in reverse at normal speed and resolution, reverse, a featureless blank screen, black, or frames played in random order, random. All are compared with a 1/300 (0.1 Hz) playing movie and significance (‘*’P<0.05, ‘***’P<0.001) was determined using Tukey’s analysis of variance method. Columns represent average and s.e. Figure 4: Larvae are visually attracted via temporal and spatial cues. Averaged crossover values of Canton S larvae crawling in a Petri dish placed over an iPad 1 playing a QuickTime movie under variable conditions. Altered movie speed, Movie speed, is from 2 × (movie recorded at 30 Hz and replayed at 60 Hz) to 1/300 × , or replayed at 0.1 Hz. The test movie was average binned, spatial resolution, down to 40 × 40, which is the same as the ‘white square movie’ in Fig. 3 . Frames were removed, temporal resolution, either every four out of five frames, 1/5 × , or every 49 out of 50, 1/50 × , and the movie was then slowed appropriately to match the live speed. In ‘other’, the movie was either played in reverse at normal speed and resolution, reverse, a featureless blank screen, black, or frames played in random order, random. All are compared with a 1/300 (0.1 Hz) playing movie and significance (‘*’ P <0.05, ‘***’ P <0.001) was determined using Tukey’s analysis of variance method. Columns represent average and s.e. Full size image Our data show that fly larvae can distinguish complex images using rudimentary visual input. Larvae are attracted to other writhing larvae and this attraction requires the visual system and can be recapitulated by playing back previously recorded writhing larvae on a computer screen. The attraction is based on both spatial and temporal cues, meaning that both motion and the quality of the image are important. Our compiled tracks of test larvae ( Figs 1b and 3a ) do not indicate a general alteration in the search strategy based on target identity and in all cases larvae average about the same amount of locomotion in the 30-min test period. This ability to visually recognize writhing in another larva may be some form of cooperative behaviour, potentially to disentangle a trapped larva or help remove an externally attached parasitic egg [7] , [8] . It may also represent opportunistic attraction to a source of food. This writhing motion is distinct from the previously described ‘rolling’ behaviour in which a kink is maintained along the larval axis and it still occurs in painless mutants [7] . Larvae are known to be attracted to burrowing larvae that make a circular motion with their posterior abdomen, not too different to the writhing reported here [3] . This previously described behaviour was proposed to be olfactory in nature when in fact it could also be visual. Two potential mechanisms allowing complex visual discrimination by simple photoreceptors are the compilation of a scanned image obtained from moving photoreceptors and the detection of moving objects in a pattern encoded by changing signals from fixed photoreceptors. In the former, the photoreceptors’ two-dimensional position would have to be encoded along with the light detected and compiled over visual sweeps. Indeed, head sweeps have been reported in insect larvae that are thought to be compiling an image [2] and fly larvae do conduct head sweeps when navigating [9] . The likely site of higher visual–spatial integration in adult flies [10] , the central complex, is present in larvae [11] . In addition, larval photoreceptors do project to the optic neuropil in a topographic manner [12] . A second approach might measure how input changes over time in a spatially fixed photoreceptor. In this scenario, the relatively slow-moving larvae can be considered as spatially fixed and thus integrating over time. A writhing larva might have just the right temporal signature of signal change to allow discrimination. Future experiments that look at both the role and timing of head movements should discriminate between these possibilities and may yield more information about how visual cues regulate behaviour. A small spot of superglue was placed on a 100-mm Petri dish lid and 4 °C cooled larvae were held on their ventral posterior side to the glue. Three larvae were placed for each spot. A water-dampened Kimwipe was placed in the base of the dish upon which was placed one foraging third instar larva that was selected from a large social group in the yeast of a standard Drosophila egg plate. The crawling larva was imaged under ambient room lighting with an iSight camera and recorded using Photobooth for 30 min. The resultant QuickTime movie was imported into ImageJ, 50-fold reduced in number of frames, first-frame subtracted from all others and z-stacked to yield a final trace. For cumulative plots in Fig. 1 , Supplementary Fig. S1 and Fig. 3 , larval position was determined every 30 s using Manual Tracker in ImageJ and registered using the central drop-off point and the larval target that is 2.5 cm left of centre. Experiments in which larvae spent more than 10 min in one spot, usually owing to injury during transfer, were not considered. Crossovers and time spent per 1/2 cm 2 was determined using Microsoft Excel and plotted using R (The R Foundation for Statistical Programming). For crossing analysis in Figs 2 and 4 , a 1 cm square was placed over the target and entries into the square counted. Dark assays were conducted in a darkroom, and the crawling larva was imaged by a 2001CIH Colour CCD Infrared Weatherproof Bullet Camera illuminated with the LED array of a second identical camera. Putty the size of a tethered larva was used in the dark experiments to mark the spots where live larvae were previously tethered. The putty was placed in an inverted ‘upper’ orientation as described in Fig. 2 . For the video target assay, a QuickTime movie ( Supplementary Movie 11 , 48 × 42 pixels) was played on a horizontally placed iPad 1 and the crossover assay was conducted above it. The minimum approach distance is about 3 mm. In preliminary experiments with a movie played on an LCD computer monitor, we also found attraction to a control white spot owing to local alterations in temperature on the monitor screen, which was not true for the iPad 1. How to cite this article: Justice, E.D. et al. The simple fly larval visual system can process complex images. Nat. Commun. 3:1156 doi: 10.1038/ncomms2174 (2012).